The complex jujube genome provides insights into fruit tree biology The jujube ( Ziziphus jujuba Mill. ), a member of family Rhamnaceae, is a major dry fruit and a traditional herbal medicine for more than one billion people. Here we present a high-quality sequence for the complex jujube genome, the first genome sequence of Rhamnaceae, using an integrated strategy. The final assembly spans 437.65 Mb (98.6% of the estimated) with 321.45 Mb anchored to the 12 pseudo-chromosomes and contains 32,808 genes. The jujube genome has undergone frequent inter-chromosome fusions and segmental duplications, but no recent whole-genome duplication. Further analyses of the jujube-specific genes and transcriptome data from 15 tissues reveal the molecular mechanisms underlying some specific properties of the jujube. Its high vitamin C content can be attributed to a unique high level expression of genes involved in both biosynthesis and regeneration. Our study provides insights into jujube-specific biology and valuable genomic resources for the improvement of Rhamnaceae plants and other fruit trees. The jujube ( Ziziphus jujuba Mill.) is the most economically important member of the Rhamnaceae, a large cosmopolitan family [1] , [2] . It is one of the oldest cultivated fruit trees in the world, with evidence of domestication dating back to 7,000 years ago [3] . It is native to China and is now a major dry fruit crop with a cultivation area of 2 million ha, the main source of income for 20 million farmers as well as a traditional herbal medicine for more than one billion people in Asia [4] . It has been introduced into at least 47 countries from temperate to tropical zones throughout the five continents and is becoming increasingly popular worldwide [5] , [6] . The jujube has a range of botanical and horticultural features [6] that gives it great potential in fruit tree molecular improvement, human health protection, and the economical development and ecological restoration of arid region. 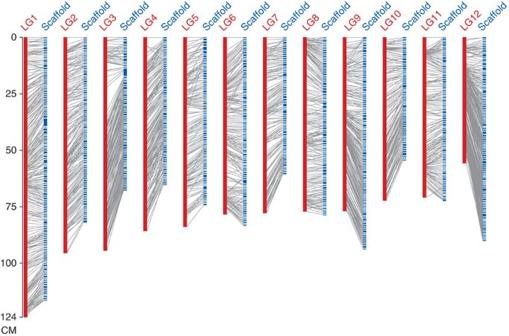Figure 1: Alignment of the genome sequence assembly with the genetic map of jujube. In total, 1,120 assembled scaffolds (blue) were anchored in the 12 linkage groups (LG1–LG12, red) using 2,213 corresponding SNP genetic markers (grey bars). The LG numbers were assigned on the basis of the estimated length of the genetic linkage groups. It is well-adapted to various biotic and abiotic stresses, especially drought and salinity ( Supplementary Table 1 ), and is considered an ideal cash crop for arid and semi-arid areas where common fruits and grain/oil crops do not grow well. 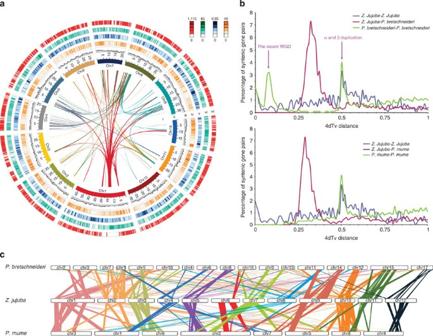Figure 2: Characterization of the jujube genome, and duplication and synteny among jujube, pear andP. mume. (a) The genomic landscape of the 12 jujube pseudo-chromosomes. All density information was counted in non-overlapping 200-kb windows. i, synteny relationship of gene blocks between pseudo-chromosomes; ii, ideograms of the 12 pseudo-chromosomes; iii, GC content density; iv, gene density; v, repeat density, estimated by counting the repeat numbers of non-redundant repeat annotation results; vi, SSR density and vii, SNP density. (b) 4DTv (fourfold synonymous third-codon transversion) value between syntenic gene pairs among the jujube, pear andP. mume. (c) Schematic representation of syntenies among the jujube (pseudo-chromosomes 1–12),P. mume(chromosomes 1–8) and pear genomes (chromosomes 1–17). Each line represents a syntenic region. Its fruit is an excellent source of vitamin C (higher than the well-known vitamin C-rich orange and kiwifruit) and sugar (25–30%, twice as high as most common fruits and even higher than sugarcane and sugar beet) [7] ( Supplementary Table 2 ). The jujube also has a very easy and quick flower bud differentiation (only ~7 days), a long flowering season lasting for 2 months, a very short period of ~6 months from planting or sowing to yielding fruits, and a very long lifecycle, even more than 1,000 productive years [3] , [6] ( Supplementary Fig. 1 ). Furthermore, jujube tree has evolved a distinct self-shoot-pruning system comprising four types of shoot namely primary shoot, secondary shoot, mother bearing shoot (MBS) and bearing shoot [6] , each of which has a very different function and developmental pattern. Primary shoot is the only normally extended shoot. Secondary shoot occurs from each node of the primary shoot and its tip dies back naturally. MBS is the branch producing bearing shoots, it is formed at each node of the secondary shoot and is extremely condensed elongating only ~1 mm per year. Bearing shoot is the only fruiting shoot, it is deciduous and drops before winter normally, which is a very uncommon trait in tree plants. This self-shoot-pruning system makes it easy to control tree size, and the diversified shoot types offers a unique model for elucidating shoot development and function. Sugar and vitamin C contents are the most common indicators of fruit quality, pruning is the most labour-consuming work of orchard management, earlier fruiting and more productive years are what farmers expect, and drought and salinity are the main abiotic stresses for fruit growing. Therefore, the aforementioned properties of the jujube are of great importance to the modern fruit production characterized by fast payback, easy management and labour-saving. In addition, the jujube is a close relative of Rosaceae (both belonging to the Rosales order in the widely accepted molecular taxonomy system of Angiosperm [8] , [9] ), the most important fruit-producing family containing a large number of leading deciduous fruit species such as apple ( Malus domestica ), pear ( Pyrus bretschneideri ), peach ( Prunus persica ), strawberry ( Fragaria vesca ) and Rubus . Consequently, the jujube could be a rich source of genes for the molecular improvement of fruit trees, and a fundamental understanding of the genetics of the jujube is crucial. So far, more than 70 plant genomes have been sequenced and assembled since the genome sequence of Arabidopsis thaliana [10] was published in 2000. However, high level of heterozygosity and repeated sequences and low content of GC are still the main obstacles for genome sequencing and assembly using the next-generation-sequencing (NGS) technology. Owing to the short read length of the NGS technology, the assembling algorithm is always based on de Bruijn graph [11] , where heterozygous locus between haploid becomes a bubble resulting in the breakdown of the final assembly at the heterozygous locus. The repeated sequences make the assembly fragmental in the similar way. Bacterial artificial chromosome-to-bacterial artificial chromosome (BAC-to-BAC) strategy was reintroduced and a few genomes have been assembled at a reasonable level [12] , [13] , [14] . We revealed not only both high heterozygosity and high density of repeated sequence but also low GC content in the jujube genome, which indicated that new method should be applied to obtain a good quality sequence for this complex genome. Knowledge of jujube genetics and genomics is very limited, and no genome-wide study (data on the genome size, heterozygosity and a completed molecular genetic linkage map) on any members of the family Rhamnaceae has so far been published, which has significantly hindered the molecular breeding, biological research and deep utilization of the jujube. In this research, we generate and analyze a high-quality genome sequence of one of the oldest and most widely cultivated Chinese jujube cultivars, ‘Dongzao’ (2 n =2 x =24), using a novel strategy integrating whole-genome shotgun (WGS) sequencing, BAC-to-BAC and a PCR-free library. We also conduct comprehensive transcriptome analyses of 15 different tissues and evolutionary comparisons with related species to identify genetic characteristics that are likely to underpin some of the most valuable traits of jujube. Our study offers a rich resource of genetic information for the breeding of jujube and the molecular improvement of other Rhamnaceae plants and fruit species. 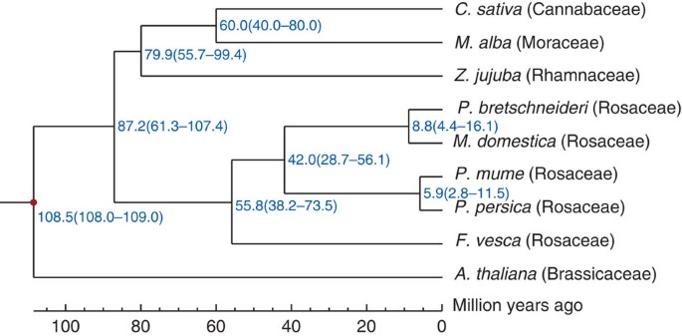Figure 3: Estimation of divergence time betweenZ. jujubaand other sequenced Rosales species. The blue numbers on the nodes are the divergence times from the present (in million years ago). The calibration time of the divergence of the malvids and fabids (108–109 million years ago) is derived from Heet al.18 Sequencing and assembly of the complex jujube genome Our analysis of the 17-mer frequency distribution based on short insert size (<1 Kbp) clean data and simulation revealed a heterozygosity of 1.90% in the jujube genome ( Supplementary Table 3 , Supplementary Fig. 2 ). 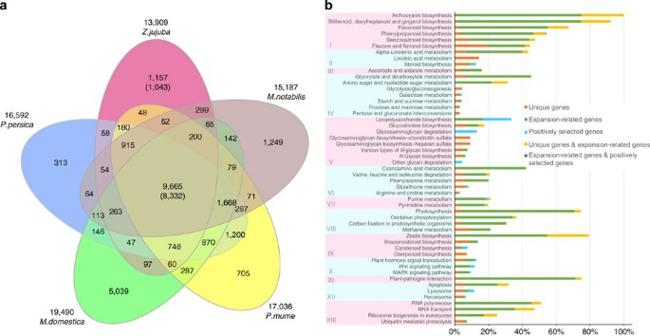Figure 4: Jujube-specific genes. (a) Venn diagram of orthologous gene families. Seven closely related Rosales species (jujube, apple, pear, strawberry, peach,P. mumeand mulberry) were used to generate the Venn diagram based on the gene family cluster analysis. The numbers in parentheses are gene families in jujube compared with all the other six related species, and the numbers without parentheses are those compared with the four species shown in the figure. (b) Ratios and distributions of jujube-specific gene sets (expansion-related genes, genes under positive selection and unique genes) in KEGG pathways. I, biosynthesis of other secondary metabolites; II, lipid metabolism; III, ascorbate and aldarate metabolism; IV, carbohydrate metabolism; V, glycan biosynthesis and metabolism; VI, amino acid metabolism; VII, nucleotide metabolism; VIII, energy metabolism; IX, metabolism of terpenoids and polyketides; X, signal transduction; XI, environmental adaptation; XII, cellular processes and XIII, genetic information processing. This is the highest degree of heterozygosity among the plants sequenced to date by NGS technology ( Supplementary Table 4 ), which is almost twice the second-highest level of heterozygosity in plants (1.02%, pear) [14] . In addition, the density of simple sequence repeats (SSRs) in the jujube genome reached 378.1 SSRs per Mb, which is 2.00 times and 2.84 times that found in its close relative species peach and apple, respectively ( Supplementary Tables 5 and 6 ) [15] , [16] . The very high level of heterozygosity, very high density of SSRs and low GC content (33.41%) ( Table 1 ) make the jujube genome a challenge for the WGS strategy using NGS technology. Table 1 Statistics of assembly and annotation for the jujube genome. Full size table A strategy combining WGS sequencing, BAC-to-BAC and WGS-PCR-free library was employed to reduce the impact of the complexity of the jujube genome. WGS was used to construct libraries of different insert sizes, ranging from 170 bp to 40 kb ( Supplementary Table 7 ). A total of 21,504 BAC clones ( Supplementary Table 8 ) were selected for sequencing at an average of 68 × coverage using the Illumina HiSeq 2000 system, representing a total of 5.86 × coverage of jujube genome size. These BAC sequences were taken as BAC end data to overcome the heterozygosity problem and to improve genome assembly. Paired-end-libraries of 170 to 800 bp were constructed and sequenced at 318 × coverage to fill in the gaps. WGS mate-pair libraries of 2, 5, 10, 20 and 40 kb were constructed and sequenced at 69 × coverage to build super scaffolds. However, parts of the genome were missing from the sequencing data owing to low GC content and the high density and even distribution of SSRs. Thus, WGS-PCR-free libraries were constructed and sequenced to reduce the bias in library construction caused by low GC content genome regions, then 30 Mb sequences were added to the final assembly. Finally, we assembled all the above sequencing data into 28,930 contigs and 5,898 scaffolds with N50 sizes of 33.95 kb and 301.04 kb, respectively, spanning 437.65 Mb of the genome sequence ( Table 1 and Supplementary Table 9 ). The assembly covered 98.6% of the jujube genome (444 Mb) estimated by our 17-mer sequence analysis ( Supplementary Table 3 , Supplementary Fig. 2 ). In jujube genome, the percentage of low GC content sequences (with GC% range from 25–30%) are much higher than that in grape vine and peach genomes ( Supplementary Fig. 3 ). To further evaluate the accuracy of the genome assembly, full-length sequences of four randomly selected BACs, later demonstrated to be located in pseudo-chromosomes 1, 2, 3 and 11 ( Supplementary Fig. 4 ), were sequenced and assembled using Sanger sequencing technology. Each BAC was aligned to three scaffolds at most, with an average coverage ratio of 98.5% ( Supplementary Table 10 and Supplementary Fig. 5 ). In addition, our assembled sequence covered >98.1% of the 1,942 published ESTs ( http://www.ncbi.nlm.nih.gov/nucest/?term=jujube , downloaded on July 2013) and 97.8% of the transcriptome sequences ( Supplementary Tables 11 and 12 ). Together, the above results indicate the high quality of our jujube genome sequence. Genome sequence anchoring and pseudo-chromosome construction To anchor the assembled genome sequences to the jujube chromosomes, we mapped the scaffolds to a high density molecular genetic map that we constructed de novo using an inter-specific population (105 progenies) between Z. jujuba (female, 2n =2 x =24) and Z. acidojujuba (male, 2n =2 x =24). Each individual in the F1 population was genotyped by restriction site-associated DNA sequencing (RAD-Seq). Sequencing reads of parents and the population are aligned to the jujube genome sequences using SOAP2 ( Supplementary Table 13 ). The final map spanned 974.01 cM for the female parent and 935.40 cM for the male parent across the 12 linkage groups, with a mean genetic distance between markers (single nucleotide polymorphisms (SNPs)) of 0.56 cM and 0.43 cM, respectively. The joint map across the 12 linkage groups was composed of 2,419 SNP markers spanning 1,020.22 cM, with a mean marker distance of 0.42 cM. Combining the assembled genome sequences and the genetic linkage groups, we constructed pseudo-molecules for each of the 12 chromosomes and ordered them on the basis of genetic length ( Supplementary Fig. 4 ). Using the mapped markers with known sequences that were uniquely aligned to the assembled scaffolds, a total of 1,120 scaffolds were anchored to the 12 linkage groups, comprising 73.56% (321.45 Mb) of the jujube genome assembly ( Fig. 1 ). Of the anchored scaffolds, 784 could be oriented (267.98 Mb, 83.37% of the total anchored sequences), suggesting high alignment accordance between the anchored genetic markers and the sequenced scaffolds. Figure 1: Alignment of the genome sequence assembly with the genetic map of jujube. In total, 1,120 assembled scaffolds (blue) were anchored in the 12 linkage groups (LG1–LG12, red) using 2,213 corresponding SNP genetic markers (grey bars). The LG numbers were assigned on the basis of the estimated length of the genetic linkage groups. Full size image Genome annotation and characterization We annotated the jujube genome by combining ab initio gene predictions, protein-based homology searches and experimental data (RNA-Seq). A total of 32,808 protein-coding genes with an average coding sequence length of 1,190 bp and 4.5 exons per gene were predicted ( Supplementary Tables 14 and 15 ). Overall, 78.26% of the gene models were predicted to contain two or more exons ( Supplementary Table 16 ), and 89.80% of the predicted proteins were supported by the RNA-Seq data ( Supplementary Table 17 ), showing the high accuracy of gene annotation. In addition, we identified a total of 410 ribosomal RNAs, 1,209 transfer RNAs, 286 small nuclear RNAs and 272 microRNAs in the jujube genome ( Supplementary Table 18 ). Tissue-specific genes and housekeeping genes were also screened in our 24 Gb of RNA-Seq data from five tissues. We found that 613, 249, 382, 553 and 184 genes were specifically expressed in the root, shoot, leaf, flower or fruit, respectively. The 16,478 genes shared by all the five tissues ( Supplementary Fig. 5 ) accounted for 81.43% of the total recorded and 50.22% of the total predicted protein-coding genes in the jujube genome. Among these shared genes, 1,818 were constitutively expressed housekeeping genes ( τ <0.07, based on the tissue specificity index [17] ), including 102 encoding ribosomal proteins and 21 encoding translation initiation factors ( Supplementary Data 1 ). We next characterized the genome by investigating genome duplication and GC content, gene density, repeat sequences, and SSR and SNP distribution along the pseudo-chromosomes ( Fig. 2 ). We identified 4.77 million SNPs in our jujube genome sequence. In total, 79.55% of them were anchored on the 12 pseudo-chromosomes, and the overall polymorphism density was 11 SNPs per kb ( Supplementary Table 19 ). The SSRs were not only present at a high density (378.1 SSRs per Mb), they were also fairly evenly distributed ( Fig. 2a , vi). We observed large regions that alternate between high and low gene density ( Fig. 2a , iv), which was also noted in peach [15] . The density of repeated sequences also reflects gene density ( Fig. 2a , iv and v). The GC content is distributed unevenly in most pseudo-chromosomes ( Fig. 2a , iii). Figure 2: Characterization of the jujube genome, and duplication and synteny among jujube, pear and P. mume . ( a ) The genomic landscape of the 12 jujube pseudo-chromosomes. All density information was counted in non-overlapping 200-kb windows. i, synteny relationship of gene blocks between pseudo-chromosomes; ii, ideograms of the 12 pseudo-chromosomes; iii, GC content density; iv, gene density; v, repeat density, estimated by counting the repeat numbers of non-redundant repeat annotation results; vi, SSR density and vii, SNP density. ( b ) 4DTv (fourfold synonymous third-codon transversion) value between syntenic gene pairs among the jujube, pear and P. mume . ( c ) Schematic representation of syntenies among the jujube (pseudo-chromosomes 1–12), P. mume (chromosomes 1–8) and pear genomes (chromosomes 1–17). Each line represents a syntenic region. Full size image We identified a total of 216.6 Mb of repeated sequences (49.49% of the assembled genome) in the jujube genome ( Supplementary Table 20 ). Among these sequences, 94.6% are transposable elements (TEs). The majority of TEs are retrotransposons (38.03% of the genome), whereas DNA transposons account for 8.08% of the genome. The most abundant (64%) retrotransposons are long-terminal repeat elements, of which 37% are Gypsy-type elements and 27% are of the Copia type ( Supplementary Table 21 ). TE content in jujube genome (46.82%), compared with its close relatives, appears to be similar to that in mulberry (47%; ref. 18 ), and higher than that in peach (37%; ref. 15 ) and P. mume (45%; ref. 19 ). About 99.41% of TEs had a divergence rate of >10% ( Supplementary Fig. 6 ), indicating that most jujube TEs are relatively ancient [18] . In total, 23,996 genes (73% of the total number of annotated genes) were allocated on the 12 pseudo-chromosomes. Self-alignment of the jujube genome sequences based on the 23,996 gene models identified 943 paralogous gene groups ( Fig. 2a,i ), indicating that the jujube genome may have undergone frequent inter-chromosome fusions and segmental duplication during its evolutionary history. Interestingly, the gene blocks located in the region from 9.20–14.68 Mb of pseudo-chromosome 1 showed obvious synteny with all other chromosomes ( Supplementary Fig. 7 ), while the very low SNP density in this block ( Fig. 2a , vii) suggests that it is highly conserved. Further analysis revealed that this block contains many genes relating to sugar metabolism and stress tolerance ( Supplementary Data 2 ). Consequently, it might be crucial for understanding the unusual characteristics of jujube. Genome comparison with closely related species To estimate speciation times, we constructed a phylogenetic tree based on single-copy genes of jujube and the seven other sequenced species of Rosales, with A. thaliana (Brassicaceae) as the outgroup ( Fig. 3 ). The results suggest a speciation time of 79.9 million years ago (Mya) for jujube and the clades of mulberry ( Morus alba , Moraceae) and Cannabis sativa (Cannabaceae), 87.2 Mya for jujube and Rosaceae (including P. bretschneideri , M. domestica , P. mume , P. persica and F. vesca ), and 108.5 Mya for jujube and A. thaliana . The speciation time is consistent with the origin time inferred from the fossil records and the recent molecular estimation [20] , [21] . Moreover, our data showed that jujube and the clade of M. alba and C. sativa diverged much earlier than the divergence of M. domestica and F. vesca in Rosaceae. Consequently, the jujube is the most ancient species among all of the sequenced species of Rosales ( Fig. 3 ). This result supports that Rhamnaceae has a long history and can be traced back to the Campanian [22] , [23] . Thus, our analysis provides new insights into the phylogeny of Rosales plants on the basis of genome-scale data. Figure 3: Estimation of divergence time between Z. jujuba and other sequenced Rosales species. The blue numbers on the nodes are the divergence times from the present (in million years ago). The calibration time of the divergence of the malvids and fabids (108–109 million years ago) is derived from He et al . [18] Full size image To further analyze the evolutionary divergence of jujube and other species, fourfold synonymous third-codon transversion (4DTv) rates were calculated ( Fig. 2b ). The 4DTv value peaked at only 0.50 in jujube, suggesting no recent whole-genome duplication occurred. The 4DTv value peaked at 0.06 and 0.50 for paralog pairs in pear, highlighting the recent whole-genome duplication and α and β duplication in this species. The orthologs between jujube and pear and between jujube and P. mume showed that 4DTv value peaked at 0.32 and 0.27, respectively, indicating that the divergence time between jujube and pear was earlier. All 4DTv values among paralogs in jujube, pear and P. mume peaked at ~0.50, indicating that the hexaploidy in these eudicots occurred at a similar time and before the split of Rhamnaceae and Rosaceae. To study the evolutionary events leading to the modern genome structure of the jujube, we analyzed the syntenic relationships among jujube, pear and P. mume (all belong to order Rosales). About 4,954 (jujube versus pear) and 5,722 (jujube versus P. mume ) orthologous genes in the jujube genome were selected. We then investigated the detailed orthologous chromosome-to-chromosome relationships between these species ( Fig. 2c ). The complicated syntenic patterns, illustrated as mosaic chromosome-to-chromosome orthologous relationships, unveiled a high degree of chromosomal evolution and rearrangements among these three species. Even so, clear syntenies could be seen among chromosomes of the three species, such as pseudo-chromosome 12 of jujube, chromosome 4 of P. mume and chromosome 17 of pear. The analysis of the synteny blocks among jujube, strawberry ( F. vesca ), peach ( P. persica ) and grape ( Vitis vinifera ) indicated that the jujube genome shares high collinearity with strawberry and peach ( Supplementary Table 22 ). To better understand jujube-specific biology, we performed comparative analyses between the jujube genome and the other six sequenced species of Rosales (apple, pear, peach, P. mume , strawberry and mulberry). We then screened these genomes based on annotated genes in the public database. Of the 32,808 protein-coding genes (13,843 gene families) in the jujube genome, 1,043 gene families are specific to jujube, and the largest number of gene clusters (11,930 families) is shared with peach ( Fig. 4a ), indicating a closer relationship between jujube and peach than between jujube and the other species analyzed. Figure 4: Jujube-specific genes. ( a ) Venn diagram of orthologous gene families. Seven closely related Rosales species (jujube, apple, pear, strawberry, peach, P. mume and mulberry) were used to generate the Venn diagram based on the gene family cluster analysis. The numbers in parentheses are gene families in jujube compared with all the other six related species, and the numbers without parentheses are those compared with the four species shown in the figure. ( b ) Ratios and distributions of jujube-specific gene sets (expansion-related genes, genes under positive selection and unique genes) in KEGG pathways. I, biosynthesis of other secondary metabolites; II, lipid metabolism; III, ascorbate and aldarate metabolism; IV, carbohydrate metabolism; V, glycan biosynthesis and metabolism; VI, amino acid metabolism; VII, nucleotide metabolism; VIII, energy metabolism; IX, metabolism of terpenoids and polyketides; X, signal transduction; XI, environmental adaptation; XII, cellular processes and XIII, genetic information processing. Full size image Expanded gene families, unique genes and genes under positive selection have important roles in plant development and evolution. The jujube-specific gene sets compared with apple, pear, strawberry, peach, P. mume and mulberry were analyzed based on the KEGG orthology pathway database, to give an insight into jujube-specific biology and adaptation. A total of 2,791 unique genes, 254 genes under positive selection and 39 expanded gene families (2,650 genes) were found and assigned to KEGG pathways ( Fig. 4b ). A further functional characterization of the above genes revealed that most of them are involved in energy metabolism, vitamin C metabolism, sugar-related metabolism and secondary metabolism. This result is consistent with the special physiological characteristics of the jujube. Genes involved in extreme accumulation of vitamin C in fruit To explore the molecular mechanism underlying the high content of vitamin C (or ascorbic acid (AsA)) in jujube fruit, we analyzed the genes encoding the key enzymes involved in all the four known AsA biosynthesis pathways and the recycling pathway during jujube fruit development. We found that those genes are involved in two of the four pathways and most of them are specific to L-galactose pathway ( Fig. 5a red part). Much fewer genes are associated with myo-inositol pathway, suggesting which maybe a compensatory pathway in jujube ( Fig. 5a blue part). Expression analyses showed that GDP-D-mannose 3,5-epimerase and GDP-L-galactose phosphorylase (two key enzymes in the L -galactose biosynthesis pathway) and monodehydroascorbate reductase ( MDHAR , the key enzyme in the AsA recycling pathway) were expressed at continuously higher levels ( Fig. 5b ). 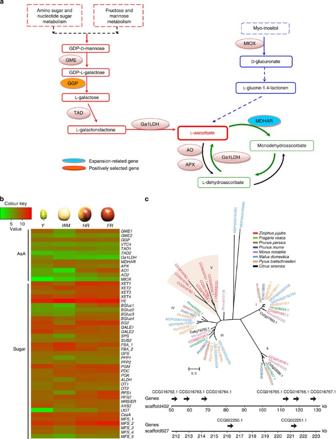Figure 5: Genes involved in sugar and AsA metabolism. (a) The pathway involved in AsA metabolism. (b) Heat map of RNA-Seq data for genes involved in AsA and sugar-related metabolism during jujube fruit ripening.Y, young fruit;WM, white mature fruit;HR, half-red fruit;FR, full red fruit. Scaled log2 expression values are shown from green to red, indicating low to high expression.GME, GDP-D-mannose 3′,5′-epimerase;GGP, GDP-L-galactose phosphorylase;VTC4, inositol-phosphate phosphatase/L-galactose 1-phosphate phosphatase;TAD,D-threo-aldose 1-dehydrogenase;Ga1LDH,L-galactono-1,4-lactone dehydrogenase;MDHAR, monodehydroascorbate reductase (NADH);AO,L-ascorbate oxidase;AP,L-ascorbate peroxidase;MIOX, inositol oxygenase;XET, xyloglucan:xyloglucosyl transferase;PE, pectinesterase;BGluc, beta-glucosidase;BG2, beta-1,3-glucanase 2;GALE, UDP-glucose 4-epimerase;SPS, sucrose-phosphate synthase;SUS2, sucrose synthase; FBA, fructose-bisphosphate aldolase;GFS, GDP-L-fucose synthase;PFP, pyrophosphate-fructose-6-phosphate 1-phosphotransferase;PGM, 2,3-bisphosphoglycerate-dependent phosphoglycerate mutase;PDC, pyruvate decarboxylase;PGK, phosphoglycerate kinase;ALDH, aldehyde dehydrogenase family 7 member A1;OT, oligosaccharyltransferase complex subunit gamma;RFS, raffinose synthase;NRS/ER, 3,5-epimerase/4-reductase;AXS2, UDP-apiose/xylose synthase;UGT, UDP-glucosyltransferase;CesA, cellulose synthase A;MFS, MFS transporter. (c) Upper part, phylogenetic analysis of theMDHARgene family in jujube and seven related species; Lower part, the location of eight MDHAR genes in two scaffolds. Figure 5: Genes involved in sugar and AsA metabolism. ( a ) The pathway involved in AsA metabolism. ( b ) Heat map of RNA-Seq data for genes involved in AsA and sugar-related metabolism during jujube fruit ripening. Y , young fruit; WM , white mature fruit; HR , half-red fruit; FR , full red fruit. Scaled log2 expression values are shown from green to red, indicating low to high expression. GME , GDP-D-mannose 3′,5′-epimerase; GGP , GDP-L-galactose phosphorylase; VTC4 , inositol-phosphate phosphatase/ L -galactose 1-phosphate phosphatase; TAD , D -threo-aldose 1-dehydrogenase; Ga1LDH , L -galactono-1,4-lactone dehydrogenase; MDHAR , monodehydroascorbate reductase (NADH); AO , L -ascorbate oxidase; AP , L -ascorbate peroxidase; MIOX , inositol oxygenase; XET , xyloglucan:xyloglucosyl transferase; PE , pectinesterase; BGluc , beta-glucosidase; BG2 , beta-1,3-glucanase 2; GALE , UDP-glucose 4-epimerase; SPS , sucrose-phosphate synthase; SUS2 , sucrose synthase; FBA, fructose-bisphosphate aldolase; GFS , GDP- L -fucose synthase; PFP , pyrophosphate-fructose-6-phosphate 1-phosphotransferase; PGM , 2,3-bisphosphoglycerate-dependent phosphoglycerate mutase; PDC , pyruvate decarboxylase; PGK , phosphoglycerate kinase; ALDH , aldehyde dehydrogenase family 7 member A1; OT , oligosaccharyltransferase complex subunit gamma; RFS , raffinose synthase; NRS/ER , 3,5-epimerase/4-reductase; AXS2 , UDP-apiose/xylose synthase; UGT , UDP-glucosyltransferase; CesA , cellulose synthase A; MFS , MFS transporter. ( c ) Upper part, phylogenetic analysis of the MDHAR gene family in jujube and seven related species; Lower part, the location of eight MDHAR genes in two scaffolds. Full size image Comparisons with the six other sequenced Rosales species at the genome level revealed that GDP-L-galactose phosphorylase is a positively selected gene and that MDHAR exhibits significant expansion in the jujube genome ( Fig. 5a,c ). Based on the phylogenetic analysis of seven Rosales species (including jujube) and one AsA-rich species (sweet orange, Citrus sinensis ) of the order Sapindales, we found that there are five major MDHAR gene subfamilies, of which subfamilies V and IV are specific to jujube and Rosaceae species, respectively ( Fig. 5c ). There are eight copies in subfamily V, which are adjacently located on two scaffolds (six in No. 402 and two in No. 627, No. 402 positioned to pseudo-chromosome 1) in the jujube genome and likely to have been generated by a tandem duplication. Interestingly, there is only one MDHAR copy (subfamilies I, II and III) in the species without recent whole-genome duplication including F. vesca (strawberry), P. persica (peach), P. mume , M. alba (mulberry), Z. jujuba (jujube) and C. sinensis (sweet orange), but there are two or more copies in the species that have undergone recent whole-genome duplication, that is, M. domestica (apple) and P. bretschneideri (pear). Collectively, our data indicate that the L-galactose pathway is the major route to AsA biosynthesis and that MDHAR contributes to AsA regeneration in jujube. Genes involved in high level accumulation of sugar in fruit To investigate the molecular mechanism underlying the high content of sugar in jujube fruit, we analyzed the genomic and RNA-Seq data and the sugar contents of fruits at four crucial development stages (young, white mature, half-red and full red). Our analysis showed that, fructose and glucose are the predominant sugars in young jujube fruits, whereas in mature fruits, sucrose and total sugar content are substantially increased, with sucrose becoming the dominant sugar ( Supplementary Table 23 ). The annotated jujube genome contains 393 genes involved in starch and sucrose metabolism, 98 involved in galactose metabolism, 67 involved in fructose and mannose metabolism, and 195 involved in amino sugar and nucleotide sugar metabolism ( Supplementary Data 3 ). Compared with other sequenced species of the order Rosales, all these gene families are expanded in jujube to some extent ( Fig. 4b , IV and V), which is consistent with the high expression patterns of these genes in jujube fruit ( Fig. 5b ). The final sugar accumulation is determined by sugar being transported from the phloem into the fruit. We found that the expression of most genes related to the major facilitator superfamily sugar transporter was enhanced in parallel with jujube fruit ripening ( Fig. 5b ). Genes involved in the distinct self-shoot-pruning system We generated and analyzed RNA-Seq data on the four types of shoot to investigate the genetic basis underlying jujube shoot biology ( Fig. 6 ). Among the four types of shoots, the number of genes differentially expressed is the smallest between primary shoot and secondary shoot, which indicates the similar metabolism of the two predominant shoots in vegetative growth. The genes related to secondary metabolism, including those involved in arginine, lipid and polyamine metabolism, were expressed at much higher levels in these two types of shoot than in bearing shoot. These results are consistent with the environmental suitability of different types of shoot. 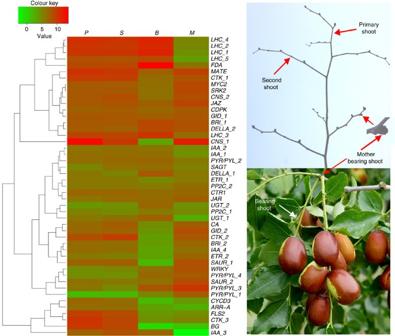Figure 6: Heat map of the normalized RNA-Seq data for genes involved in shoot development. P, primary shoot;S, secondary shoot;M, mother bearing shoot;B, bearing shoot. Scaled log2 expression values are shown from green to red, indicating low to high expression, respectively.LHC, light-harvesting complex;FDA, fructose-bisphosphate aldolase;MATE, multidrug resistance protein;CTK, cytokinin receptor;MYC2, transcription factor MYC2;SRK2, serine/threonine-protein kinase SRK2;CNS, chitinase;JAZ, jasmonate ZIM domain-containing protein;CDPK, calcium-dependent protein kinase;GID, gibberellin receptor;BRI, protein brassinosteroid insensitive;DELLA, DELLA protein;IAA, auxin-responsive protein;PYR/PYL, abscisic acid receptor PYR/PYL family;SAGT, pathogen-inducible salicylic acid glucosyltransferase;ETR, ethylene receptor;PP2C, protein phosphatase 2C;CTR1, serine/threonine-protein kinase CTR1;JAR, jasmonic acid-amino synthetase;UGT, UDP-glucosyltransferase;CA, Ca2+-transporting ATPase;SAUR, SAUR family protein;WRKY, WRKY transcription factor;CYCD3, cyclin D3; ARR-A, two-component response regulator;FLS2, LRR receptor-like serine/threonine-protein kinase FLS2;BG, beta-glucosidase. The figures on the right indicate different types of shoot. Figure 6: Heat map of the normalized RNA-Seq data for genes involved in shoot development. P , primary shoot; S , secondary shoot; M , mother bearing shoot; B , bearing shoot. Scaled log2 expression values are shown from green to red, indicating low to high expression, respectively. LHC , light-harvesting complex; FDA , fructose-bisphosphate aldolase; MATE , multidrug resistance protein; CTK , cytokinin receptor; MYC2 , transcription factor MYC2; SRK2 , serine/threonine-protein kinase SRK2; CNS , chitinase; JAZ , jasmonate ZIM domain-containing protein; CDPK , calcium-dependent protein kinase; GID , gibberellin receptor; BRI , protein brassinosteroid insensitive; DELLA , DELLA protein; IAA , auxin-responsive protein; PYR/PYL , abscisic acid receptor PYR/PYL family; SAGT , pathogen-inducible salicylic acid glucosyltransferase; ETR , ethylene receptor; PP2C , protein phosphatase 2C; CTR1 , serine/threonine-protein kinase CTR1; JAR , jasmonic acid-amino synthetase; UGT , UDP-glucosyltransferase; CA , Ca 2+ -transporting ATPase; SAUR , SAUR family protein; WRKY , WRKY transcription factor; CYCD3 , cyclin D3; ARR-A, two-component response regulator; FLS2 , LRR receptor-like serine/threonine-protein kinase FLS2; BG , beta-glucosidase. The figures on the right indicate different types of shoot. Full size image In MBS, the genes involved in abscisic acid (ABA) synthesis, such as the PYR/PYL genes, were much more highly expressed than in other shoot types, which might be a genetic basis of the extreme slow growth of MBS and the deciduous habit of bearing shoot attached on MBS. And the genes involved in porphyrin and chlorophyll metabolism were dramatically downregulated in the MBS, illustrating the decline in photosynthesis in this type of shoot. In bearing shoot, the genes related to photosynthesis, such as those in the light-harvesting chlorophyll binding protein gene family and those involved in carbohydrate metabolism, were expressed at much higher levels than in all the other three shoot types, and the genes responsive to brassinosteroids and cytokinins were expressed at much lower levels in bearing shoots. The gene expression profiles meet the needs of its fruiting function and deciduous habit. One of the more interesting things is that bearing shoots are normally deciduous, but could become lignified and persistent (not drop in the winter) in case they are extremely vigorous ( Supplementary Fig. 9 ). The genes involved in plant hormone signal transduction were expressed in patterns, suggesting that they play key roles in this process. Small auxin-up RNA, cyclin D3 and two-component response regulator ARR-A family, which are responsive to auxin, brassinosteroids and cytokinins, respectively, were much more highly expressed in lignified bearing shoots ( Supplementary Table 24 ). However, genes responsive to ethylene and ABA, such as ABA responsive element binding factor, serine/threonine-protein kinase SRK2 and ethylene-responsive transcription factor 1, were more strongly expressed in deciduous bearing shoots ( Supplementary Table 24 ). In addition, genes responsive to jasmonic acid were expressed at lower levels in deciduous bearing shoots than in persistently lignified ones ( Supplementary Table 24 ), indicating weaker stress resistance of the deciduous bearing shoot. Genes involved in the adaptation to abiotic/biotic stress Gene Ontology annotation of the jujube-specific gene families showed that some of them may take part in defence and stress responses ( Fig. 4b , XI and Supplementary Data 4 ). The number of the gene families functionally annotated as ‘response to stress’ reaches up to 854. Arginine metabolism plays an important role in plants’ perception and adaptation to environmental disturbances, and many jujube-specific genes are also enriched in this pathway ( Fig. 4b , VI). The genes responding to osmotic stress are expressed at very high levels at all stages of fruit development, which is consistent with jujube's salt tolerance and drought resistance ( Supplementary Table 25 ). Chitinases are pathogenesis related proteins that are induced by biotic and abiotic stress in plants [24] , [25] . The high expression of chitinases in jujube shoots may contribute to its high stress tolerance ( Supplementary Table 26 ). There are 13 genes encoding homologues of autophagy-related protein 9 in the jujube genome, and only 1–2 in the other 6 related species of Rosales ( Supplementary Table 27 ). Autophagy has important roles in various cellular functions [26] . Specifically, in immunity, the stimulation of autophagy in infected cells helps the cells to degrade and eliminate intracellular pathogens. Therefore, autophagy may play important roles in jujube's defence responses. Resistance (R) proteins function mainly in biotic stress responses, and they possess both a nucleotide-binding site (NBS) and a leucine rich repeat (LRR). Enrichment analyses of both IntrePro domains and gene ontology terms showed that the 849 R genes in jujube could be classified into 7 groups: CC-NBS-LRR, CC-NBS, LRR-RLK, NBS-LRR, NBS, TIR-NBS-LRR and TIR-NBS. The CC-NBS-LRR group (115 genes) was the most abundant among the 11 sequenced species from diversified taxa ( Supplementary Table 28 ). A large number of R genes (140, 16%) are scattered throughout chromosome 9, indicating that this chromosome is an important candidate target for further research on disease resistance of jujube. Moreover, 17% of jujube genes with a nucleotide-binding adaptor shared by APAF-1, R proteins and CED-4 domain are unique genes or positively selected genes, which suggests that the function of disease resistance has been reinforced during jujube evolution ( Supplementary Table 29 ). High rate of heterozygosity remains a particular challenge for de novo assembly [27] . However, most perennial tree species are highly heterozygous [28] , [29] , [30] , and it is complicated and time-consuming to obtain their double haploid or pure line materials of very low heterozygosity. The jujube genome was characterized as high in heterozygosity, high in density of SSRs and low in GC content. High level of heterozygosity will fragment the assembly of diploid genome sequenced only using the NGS technology or WGS strategy, whereas BAC-to-BAC strategy could avoid this problem via sequencing and assembling of each haploid BAC sequence. Due to the high SSR density and low GC content of jujube genome, some genomic regions were missed in the WGS-PCR sequencing. To retrieve such sequences, WGS-PCR-free library was constructed and sequenced, and 30 Mb sequences were added to the final assembly. The finished assembly covers 98.6% of the estimated jujube genome, >98% of the de novo transcriptome sequence and 1,942 published ESTs, and it shows an overall identity of 98.5% with four randomly chosen BAC sequences. Consequently, this integrated strategy provides a good solution for assembling the complex jujube genome based on the most widely used NGS technology nowadays. Our genomic and RNA-Seq analyses of the jujube offers some insights into the molecular mechanisms underlying the extreme accumulation of vitamin C and sugar in fruit, the distinct self-shoot-pruning system and the outstanding tolerance to abiotic/biotic stress, which are what the main breeding objectives of fruit trees. Compared with orange and kiwifruit, two well-known vitamin C-rich fruits with expansion and high expression of genes involved in the biosynthesis and recycling of vitamin C (refs 31 , 32 ), respectively, the gene involved in both the biosynthesis and the recycling of vitamin C are enhanced in jujube ( Fig. 5 ). This is the first report on such a kind of accumulation mechanism of vitamin C in fruit to our knowledge, which might elucidate why the vitamin C content of jujube is much higher than that in orange and kiwifruit ( Supplementary Table 2 ). This study indicates that the jujube would be a useful source of genes of fruit nutrition, self-shoot-pruning and stress tolerance for introduction into other fruit crops. To better understand and use the specific traits of jujube, more studies should be carried out integrating further genomic and transcriptome analysis, physiological analysis and field experiment. The newly obtained high-quality genome sequence and gene information linked to its valuable biological features, a relatively small genome of 444 Mb similar to rice (466 Mb) and diploid inheritance with 12 pairs of chromosomes as in rice, coupled with its suitable biological properties including very short generation time, relatively small tree size, easy and quick flower bud differentiation, long flowering season, ease of vegetative propagation and cultivation, and a well-established in vitro regeneration system [33] , [34] , [35] , will enable the use of the jujube as a potential reference genomic system for deciduous fruit trees. WGS sequencing and BAC sequencing Genomic DNA was extracted from in vitro grown Z. jujuba Mill. ‘Dongzao’ plantlets. Paired-end and mate-pair Illumina WGS libraries were constructed with multiple insert sizes (170 bp to 40 kb) according to the manufacturer’s instructions (Illumina). For each short insert size (170, 250, 500 and 800 bp) library construction about 5 μg genomic DNA was used, and for large insert size (2, 5, 10, 20 and 40 Kb) library construction 20~60 μg DNA was used. Genomic DNA was fragmented, linked to adapters and extracted at specific size after agarose gel electrophoresis. For large insert size, first, fragments were biotin-labelled and circularized after size selection, sheared and enriched by magnetic beads (Invitrogen). Purified DNA was amplified by PCR, cloned to vector to yield 20 libraries for Illumina Hiseq 2000 sequencing. We obtained 188.86 Gb raw WGS sequencing data. In the raw data filtering process, several heuristic rules were applied: (1) we removed reads with >2% Ns or with poly-A structure; (2) we removed reads with ≥40% low quality bases for short insert size libraries and ≥60% for large insert size libraries; (3) we removed reads containing adapters; (4) we removed paired reads with mutual overlaps; (5) we removed PCR duplicates. After filtering, 109.88 Gb high-quality data were retained, representing 249.72 × genome coverage. To overcome the key issue of high heterozygosity, high repeat content, we also constructed BAC libraries with insert fragment size of 120 kb length. A total of 21,504 BAC clones were randomly selected to extract plasmids. For each clone, unique index primer and adapter index were linked to fragment end, and a 500 bp insert size library was constructed and used for Illumina sequencing to a coverage depth of ~5.8 × . A pooling of 2,688 libraries (equal to 28 × 96-well plates) was sequenced in one lane, totally 21,504 libraries were sequenced in eight lanes to generate 177.17 Gb raw data for BAC sequencing ( Supplementary Table 8 ). De novo genome assembly The short insert size library data were corrected by correct_error programme in the SOAPdenovo [11] software package, which changed error bases in low frequency K-mers to form high frequency K-mers. The jujube genome was de novo assembled using a hierarchical assembly strategy [36] along with WGS strategy. We assembled WGS sequencing data using SOAPdenovo-2.04 (ref. 11 ) software with K-mer value set as 87. The procedure included three steps: (1) construct de Bruijn graph using the short insert size data; (2) construct scaffold by aligning reads onto the contigs and (3) fill gaps by local assembly through mapping reads to flanking sequences of gaps. For BAC sequencing data, we split each BAC library data by index sequences in SOAPdenovo-2.04 (ref. 11 ) software to assemble each BAC clone. We combined the above WGS assembled sequences with the above assembled BAC sequences based on the overlap information by Rabbit [37] , and then used the paired-end relationships of the large insert size sequencing data to link the scaffolds/contigs into super-scaffold sequence using SSPACE-v1.1 (ref. 38 ). We filled gaps by GapCloser v1.10 programme in the SOAPdenovo [11] software package. To overcome the problems associated with low GC content of the jujube, PCR-free libraries were also constructed and sequenced. RAD-seq for genetic map construction The mapping population consisted of 105 inter-specific hybrids from a cross between Z. jujuba Mill. ‘JMS2’ and Z. acidojujuba Cheng et Liu ‘Xing 16’. Each individual in the F1 population was genotyped with RAD-seq. The paired-end RAD reads was mapped by SOAP2 (ref. 39 ). Based on the alignment result, the RAD-based SNP calling was done by SOAPsnp [40] . Two heterozygous SNP alleles or one heterozygous and one homozygous SNP allele between two parents were treated as potential SNP markers if the following criteria were satisfied: parents:sequencing depth ≥10, base quality ≥25, copy number ≤1.5; progenies:sequencing depth ≥6, base quality ≥20, copy number ≤1.5. The ratio of marker segregation was calculated by χ 2 -test. Markers showing significantly distorted segregation ( P -value < 0.01) were excluded from the map construction. The double pseudo-test cross strategy was applied [41] . Linkage analysis was performed for markers present at least 85% using JoinMap 4.0 software with CP population type codes [42] . An logarithm (base 10) of odds (LOD) score of 6.0 was initially set as the linkage threshold for linkage group identification. Twelve linkage groups that had the same number of jujube chromosomes were formed at a LOD threshold of 6.0 and ordered using the regression mapping algorithm. Linkage between markers, recombination rates and map distances were calculated using the Kosambi mapping function and the regression mapping algorithm with a recombination frequency threshold of 0.5. The mapping position of SNP markers were first aligned to the scaffolds and scaffolds with only one SNP marker could be anchored but not oriented owing to a lack of markers. Finally, we scanned all SNP markers to construct the linkage groups and to anchor scaffolds to chromosomes. Repeat annotation Repetitive elements were identified by Repbase-based method [43] , de novo approach and TRF [44] software. We searched for repeats using RepeatMasker [45] and RepeatProteinMask [45] software against Repbase database, identifying TEs at DNA and protein level. Also, we employed Piler [46] , RepeatScout [47] , and LTR-FINDER [48] programmes to build the de novo repeat libraries and we ran RepeatMasker against the de novo library to find and classify the repeats. Gene prediction We used homology-based and de novo methods, as well as RNA-seq data, to predict genes in the Z. jujuba genome. For homology-based gene prediction, protein sequences from six other plant species ( C. sinensis , M. domestica , P. trichocarpa , G. max , P. persica and V. vinifera ) were initially mapped onto the Z. jujuba genome using TBLASTN [49] ( E -value<1e−5), and the homologous genome sequences were aligned against the matching proteins using GeneWise [50] for accurate spliced alignments. Next, we used the de novo gene prediction methods Augustus [51] and GenScan [52] . We then integrated the homologues and those from de novo approaches using GLEAN [53] to produce a consensus gene set. In addition, we aligned all the RNA-seq reads to the reference genome using TopHat [54] and predicted the open reading frames (ORFs)s from the resulting data. Finally, we combined the GLEAN set with the gene models produced from RNA-seq to generate a high confidence gene set. We did functional gene annotation by BlastP alignment to KEGG [55] , SwissProt [56] and TrEMBL [56] databases. Motifs and domains were determined by InterProScan [57] against protein databases such as ProDom, PRINTS, Pfam, SMART, PANTHER and PROSITE, and Gene Ontology [58] was obtained from the corresponding InterProScan entries. Gene family clusters The protein-coding genes from seven Rosales species&#8232;( F. vesca , P. persica , P. mume , M. notabilis , M. domestica , P. bretschneideri and C. sativa ) and A. thaliana were downloaded from NCBI. The longest ORF was chosen to represent each gene, and ORF of genes encoding <50 amino acids were filtered out. The OrthoMCL [59] method was then used to cluster all the genes into paralogous and orthologous groups on the BLASTP alignment with pairwise comparison strategy ( E -value ≤1e−5). Speciation time estimation The phylogenetic tree of eight species including jujube was constructed. The divergence time between jujube and seven other sequenced species of Rosales ( A. thaliana as the outgroup) was estimated using MrBayes [60] and the MCMCtree programme was implemented in the Phylogenetic Analysis by Maximum Likelihood (PAML) [61] software package. Calibration times was obtained from the TimeTree database ( http://www.timetree.org/ ). Transcriptome sequencing and analysis Total RNA was extracted from 15 samples (root, primary shoot, secondary shoot, MBS, bearing shoot, leaf, flower, young fruit, white mature fruit, half-red fruit and full red fruit of ‘Dongzao’, deciduous and lignified bearing shoots of ‘Dongzao’ and ‘Lizao’ (four samples)). The deciduous and lignified bearing shoots were sampled on 26 July 2013, the stage at which we could confirm the shoots are deciduous or lignified according to the morphological characters. RNA-seq libraries were constructed to sequence the transcriptome of each sample. RNA-seq libraries were sequenced on an Illumina Genome Analyzer platform. The resulting reads were aligned to the Z. jujuba genome sequences using TopHat [54] . After alignment, the count of mapped reads from each sample was derived and normalized to reads per kilobase of exon per million reads mapped for each predicted transcript using the Cufflinks [54] package. In addition to conducting the analysis described above for the Z. jujuba transcriptome, we further assembled all reads from Z. jujuba using the Trinity [62] package to evaluate the gene region coverage ratio. Jujube-specific gene set analysis We obtained three types of specific gene set for jujube (expansion-related genes, positively selected genes and unique genes) from seven Rosales species ( Z. jujuba , F. vesca , P. persica , P. mume , M. notabilis , M. domestica and P. bretschneideri ). To obtain the jujube unique gene families, we clustered gene families of the seven sequenced Rosales plant genomes. The genes from these genomes were collected and aligned to each other using BLASTP. Pairwise protein sequence similarity was used as the distance for clustering genes. To detect genes evolving under positive selection in jujube, we used gene clustering of the seven Rosales species to identify 1,420 single-copy orthologous genes and used the optimized branch-site model [63] to identify 254 genes that are positively selected in Z. jujuba . To detect expansion gene categories (SwissProt, KEGG and InterPro), we annotated the gene functions of the seven sequenced Rosales species genes and analyzed over-represented categories. Each domain of the three categories (SwissProt, KEGG and InterPro) was retrieved from the seven Rosales species, and examples in which the abundance differed between jujube and all six other species were identified by applying Fisher’s Exact test (significance was assumed if P <0.05). Fruit sugar analysis The experiment was designed as a complete randomized block with three replicates, and four plants were used in each replicate. All samples (each 0.5 kg fruits) were picked from Z. jujuba ‘Dongzao’ at four developing stages including young (60 days after fruit set), white mature (90 days after fruit set), half-red (105 days after fruit set) and full red (120 days after fruit set) in National Jujube Germplasm Repository, Taigu, China. After drying overnight at 60 °C in the presence of silica gel, all samples were milled to powder. For each sample, 1 g of powder was transferred to a 50 ml volumetric flask and diluted to 40 ml with water of ultrapure grade. The flask was sonicated for 1 h at 80 °C. After cooling to room temperature, the mixture was diluted to the volume. The extracts were filtered through filter paper and a fraction of the filtrate was filtered through a 0.45 μm membrane filter. An HPLC system (Agilent 1200 HPLC Series, Waldbronn, Germany) equipped with a quaternary pump system, a refractive index detector (G1362A) was used for sucrose, glucose and fructose analysis [64] . Total sugar was determined by the anthrone method [65] . Three replicates were done for each sample and each analysis as well. Accession codes: The Jujube genome data has been deposited at DDBJ/EMBL/GenBank under the accession code JREP00000000. Sequence reads of transcriptome sequencing have been deposited in NCBI sequence read archive (SRA) under the accession code SRP046073. How to cite this article : Liu, M.-J. et al . The complex jujube genome provides insights into fruit tree biology. Nat. Commun. 5:5315 doi: 10.1038/ncomms6315 (2014).